Discovery of the action of a geophysical synchrotron in the Earth’s Van Allen radiation belts Although the Earth’s Van Allen radiation belts were discovered over 50 years ago, the dominant processes responsible for relativistic electron acceleration, transport and loss remain poorly understood. Here we show evidence for the action of coherent acceleration due to resonance with ultra-low frequency waves on a planetary scale. Data from the CRRES probe, and from the recently launched multi-satellite NASA Van Allen Probes mission, with supporting modelling, collectively show coherent ultra-low frequency interactions which high energy resolution data reveals are far more common than either previously thought or observed. The observed modulations and energy-dependent spatial structure indicate a mode of action analogous to a geophysical synchrotron; this new mode of response represents a significant shift in known Van Allen radiation belt dynamics and structure. These periodic collisionless betatron acceleration processes also have applications in understanding the dynamics of, and periodic electromagnetic emissions from, distant plasma-astrophysical systems. It is now generally accepted that the acceleration processes generating the relativistic electrons in the outer Van Allen radiation belts act inside the Earth’s magnetosphere. However, the processes which are most geo-effective in energizing the belts under differing solar wind and geomagnetic conditions remain hotly debated [1] , [2] , [3] , [4] . Prominent candidates for dominant acceleration processes include resonance with waves in the extremely low frequency/very low frequency band such as lower band whistler mode chorus [2] , [4] , [5] , which violate the first adiabatic invariant, and interactions with ultra-low frequency (ULF) waves which violate the third invariant while conserving the first [3] , [6] , [7] , [8] , or some combination thereof [9] . Observations of local peaks in electron phase space density have suggested the potential dominance of lower band chorus acceleration [2] , although such signatures may also be generated by short wavetrain coherent ULF waves [10] . Fast solar wind speeds [11] , [12] , enhanced ULF wave power [7] , [8] , [13] , and enhancements in radiation belt electron flux are also well correlated. Typically, partly because of the paucity of observed discrete frequency modulations in MeV electron flux, the ULF wave–electron interaction is assumed to be stochastic and modelled using radial diffusion theory [3] . Narrow-band coherent ULF waves can accelerate particles proportional to time through drift resonance, whereas diffusive radial transport is slower and acts as the square root of time [10] , [14] . Determining the importance of coherent ULF acceleration and transport is hence important for understanding radiation belt morphology and dynamics; coherent acceleration being analogous to particle acceleration in synchrotron machines. In this Article, we present data and analysis of coherent interactions between ULF waves and relativistic electrons in the Van Allen belts. Using data from the Combined Release and Radiation Effects Satellite (CRRES) and from the recently launched NASA Van Allen Probes mission, we present observations of this coherent ULF wave acceleration process representing the action of a process analogous to a geophysical synchrotron on a planetary scale. 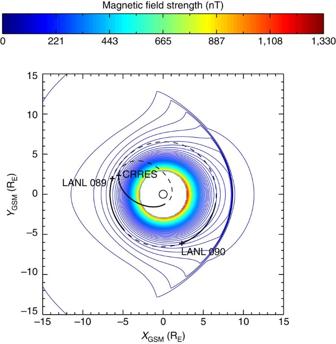Figure 1: Satellite orbits on 24 March 1991. Orbits of the CRRES and LANL 1990-095 (LANL 090) and LANL 1989-046 (LANL 089) in the GSM equatorial plane during a coherent large amplitude ULF wave–particle interaction from 10:00–14:00 UT on 24 March 1991. Overplotted are contours of constant magnetic field strength from the Tsyganenko and Sitnov152004 magnetic field model (using solar wind dynamic pressure of 10 nPa, interplanetary magnetic fieldBy=8 nT,Bz=−33 nT andDst=−250 nT) in the GSM equatorial plane. These define the unperturbed path which 90° pitch angle electrons follow along adiabatic gradient-curvature drift paths. CRRES observations and modelling Figure 1 shows satellite locations during a coherent large amplitude ULF wave–particle interaction from 10:00–14:00 UT on 24 March 1991. The 24 March 1991 was a truly remarkable day for radiation belt physics discovery, since around 8 h earlier following a sudden storm commencement at 3:41 UT a new inner zone electron radiation belt was formed in only a few minutes by a single shock passage through the magnetosphere [16] . Figure 1: Satellite orbits on 24 March 1991. Orbits of the CRRES and LANL 1990-095 (LANL 090) and LANL 1989-046 (LANL 089) in the GSM equatorial plane during a coherent large amplitude ULF wave–particle interaction from 10:00–14:00 UT on 24 March 1991. Overplotted are contours of constant magnetic field strength from the Tsyganenko and Sitnov [15] 2004 magnetic field model (using solar wind dynamic pressure of 10 nPa, interplanetary magnetic field B y =8 nT, B z =−33 nT and Dst =−250 nT) in the GSM equatorial plane. These define the unperturbed path which 90° pitch angle electrons follow along adiabatic gradient-curvature drift paths. Full size image The unfiltered ULF wave magnetic field from 10:00–14:00 UT from the Oulu (OUL) station shown in Fig. 2 (top panel) is remarkably monochromatic, having large amplitudes ~400nT p–p at L =4.5 and the characteristics of a driven field line resonance (FLR) standing along the background magnetic field, as measured by European ground-based magnetometers in the local noon sector [17] . Typically FLRs have maximum power in the auroral zone around L ~7–9 (ref. 18 ). However, in this case large amplitude monochromatic ULF wave fields peaked in the heart of the outer Van Allen belt. Likely the waves are a magnetospheric cavity oscillation, excited in the near-noon sector by dynamic pressure fluctuations in the solar wind (see Lee et al. [17] for further discussion). 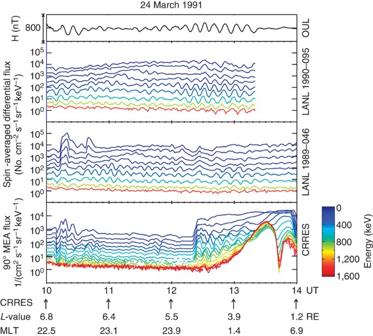Figure 2: Ground-based and satellite observations from 24 March 1991. From top to bottom: H-component magnetic field from Oulu (OUL) station (61.4°N, 106.1°E, geomagnetic), omni-directional differential flux from the SOPA instrument on the geosynchronous LANL 1990-095 and LANL 1989-046 satellites, and 90° pitch angle differential flux from CRRES MEA, respectively, from selected energy channels. The magnetic L-shells and magnetic local time (MLT) of the CRRES satellite are shown in the axis label; L-shell labels dipole magnetic field lines via the geocentric distance to their equatorial crossing point in units of Earth radii. Figure 2: Ground-based and satellite observations from 24 March 1991. From top to bottom: H-component magnetic field from Oulu (OUL) station (61.4°N, 106.1°E, geomagnetic), omni-directional differential flux from the SOPA instrument on the geosynchronous LANL 1990-095 and LANL 1989-046 satellites, and 90° pitch angle differential flux from CRRES MEA, respectively, from selected energy channels. The magnetic L-shells and magnetic local time (MLT) of the CRRES satellite are shown in the axis label; L-shell labels dipole magnetic field lines via the geocentric distance to their equatorial crossing point in units of Earth radii. Full size image The imprint of the coherent ULF wave can be seen globally throughout the electron radiation belt in the omni-directional flux from the SOPA instrument on two Los Alamos (LANL) geosynchronous satellites [19] , and differential flux from the MEA [20] (Medium Energy-A electron spectrometer) instrument on the CRRES [21] in-bound in the midnight-dusk local time sector ( Fig. 1 ). The panels in Figs 2 and 3a show ULF wave and electron time series and power spectra, respectively. The second panel of Figs 2 and 3a shows clear ULF modulation of electron flux at the same frequency as the ULF waves seen on the ground at the Oulu (OUL) magnetometer station (panel a). Note that the waves seen at OUL exercise a non-local impact on the electrons, which is seen by the satellite energetic particle detectors elsewhere around the drift orbit. LANL 1990-095, in the pre-noon local time sector, sees modulation peaking in the 315–500 keV energy channel with clear 180° phase change across energy. As the gradient-curvature drift frequency of the electrons increases with energy, the phase change in the modulation as a function of energy is that expected from what is effectively the response of harmonic oscillators with different (drift) frequencies in response to a coherent single frequency ULF wave driver through drift resonance [6] , [10] , [13] , [14] . This is an expected but previously unreported observational ‘smoking gun’ signature of ULF drift resonance with relativistic (>~500 keV) electrons in the Van Allen belts [13] . 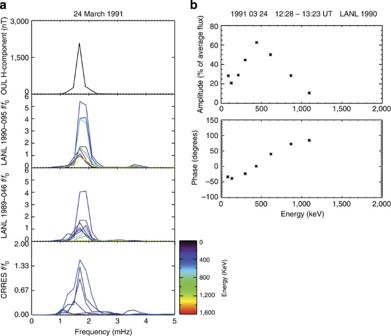Figure 3: Energetic particle power spectra on 24 March 1991. (a) Power spectra for the data shown inFig. 2, where for the particle data power spectra are normalized with respect to the background fluxf0in each channel and colour represents the energy channel of each trace. (b) Amplitude and phase of the 1.7 mHz flux modulation as a function of energy from the LANL 1990-095 SOPA data. Figure 3b confirms the resonant amplitude and phase characteristics using complex demodulation [22] analysis applied to the LANL 1990-095 data. The CRRES data (shown in ref. 23 ) indicate a similar resonant response, but with a larger phase change likely due to crossing ULF resonance islands [24] in-bound to lower-L. Note the ULF advection of spatial gradients across the satellite can create flux modulation, but with energy-independent phase [13] . Figure 3: Energetic particle power spectra on 24 March 1991. ( a ) Power spectra for the data shown in Fig. 2 , where for the particle data power spectra are normalized with respect to the background flux f 0 in each channel and colour represents the energy channel of each trace. ( b ) Amplitude and phase of the 1.7 mHz flux modulation as a function of energy from the LANL 1990-095 SOPA data. 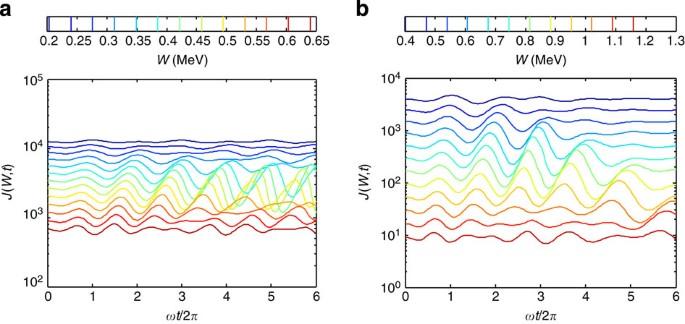Figure 4: ULF wave–particle interaction simulation for 24 March 1991. Model 90° pitch angle differential flux under ULF drift resonance with a discrete frequency 1.67 mHz FLR atL=4.3 withm=2 at (a) geosynchronous orbit (appropriate for LANL), and (b) along a virtual CRRES trajectory. Note that an azimuthally standing wave, for example, near noon (cf. the OUL magnetic field data) produces similar results as only the eastward travelling component of the oppositely directed propagating modes which comprise a standing mode will be drift-resonant with the electrons. Full size image Figure 4 shows results from tracing 90° pitch angle electrons using Liouville’s theorem with the Degeling and Rankin model [24] . Resonant particles experience ULF wave drift resonance ω = m·ω d , where ω is the wave frequency, ω d is the particle drift frequency and m is the (dimensionless) azimuthal wavenumber under the action of a 1.67 mHz FLR at L =4.3 with m =2 in a dipole field. An initial Gaussian spectrum with an electron temperature of 0.1 MeV is assumed, with background radial gradients defined by conservation of the first adiabatic invariant. The modelled flux response at geosynchronous orbit ( Fig. 4a ), and along model CRRES trajectory ( Fig. 4b ), are in excellent agreement with the observational data in Fig. 2 . The sharp rise in the CRRES data around 12:20 UT in Fig. 2 might suggest a particle injection. However, the energy-dependent phase response [13] in the multi-satellite data ( Figs 2 and 3 ) and modelling ( Fig. 4 ) provide the ‘smoking gun’ indicating a coherent and monochromatic drift-resonant ULF wave interaction as CRRES enters closed drift shells in the outer belt. Figure 4: ULF wave–particle interaction simulation for 24 March 1991. Model 90° pitch angle differential flux under ULF drift resonance with a discrete frequency 1.67 mHz FLR at L =4.3 with m =2 at ( a ) geosynchronous orbit (appropriate for LANL), and ( b ) along a virtual CRRES trajectory. Note that an azimuthally standing wave, for example, near noon (cf. the OUL magnetic field data) produces similar results as only the eastward travelling component of the oppositely directed propagating modes which comprise a standing mode will be drift-resonant with the electrons. Full size image NASA Van Allen Probe observations The launch of the two satellite NASA Van Allen Probes (formerly named the Radiation Belt Storm Probes (RBSP)) mission into near-equatorial geo-transfer orbit from Cape Canaveral on 30 August 2012 heralds a new era in radiation belt physics [25] . With apogee near L =6, and carrying a payload of a comprehensive suite of particle and fields sensors designed to study the Earth’s radiation environment, the Van Allen Probes offer a new opportunity for multi-point studies of the dynamics of the radiation belts. Although the coherent ULF acceleration seen in the CRRES data in Figs 2 and 3 is striking, previous satellite data sets suggested that such modulations were relatively rare, had limited impact across only a narrow range of energies, and only lasted for short times. The unprecedented energy resolution and cleanliness of the Energetic Particle Composition and Thermal Plasma Suite (RBSP-ECT) data, however, reveal an outer electron belt which very often displays ULF flux modulation. 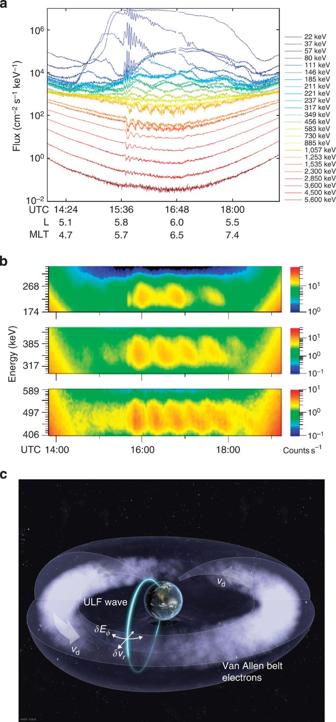Figure 5: Van Allen Probe Observations on 31 October 2012. (a) Spin-averaged differential electron flux from the MagEIS and Relativistic Electron Proton Telescope instruments in the ECT instrument suite on the RBSP-A satellite from the Van Allen Probes mission on 31 October 2012. (b) Higher resolution histogram data from MagEIS from 3 selected channels showing the long period flux modulation. (c) Schematic diagram showing the generation of drift-resonant ULF flux modulation through drift-phase bunching. Flux tube ULF radial motions,δvr, generate electric fields δEϕwhich do work on the electrons at a rate. A discrete frequency FLR, standing along the background magnetic field between reflecting ionospheres, and resulting azimuthal structure of eastward drifting ULF modulated relativistic electron flux are shown schematically. Figure 5a shows spin-averaged, differential electron flux data from the Magnetic Electron Ion Spectrometer [26] (MagEIS) and Relativistic Electron Proton Telescope [27] instruments in the RBSP-ECT suite from probe A ( L =6.01, MLT=5.94 at 16:00 UT), from 31 October 2012. Figure 5: Van Allen Probe Observations on 31 October 2012. ( a ) Spin-averaged differential electron flux from the MagEIS and Relativistic Electron Proton Telescope instruments in the ECT instrument suite on the RBSP-A satellite from the Van Allen Probes mission on 31 October 2012. ( b ) Higher resolution histogram data from MagEIS from 3 selected channels showing the long period flux modulation. ( c ) Schematic diagram showing the generation of drift-resonant ULF flux modulation through drift-phase bunching. Flux tube ULF radial motions, δv r , generate electric fields δ E ϕ which do work on the electrons at a rate . A discrete frequency FLR, standing along the background magnetic field between reflecting ionospheres, and resulting azimuthal structure of eastward drifting ULF modulated relativistic electron flux are shown schematically. Full size image Following a sharp dynamic pressure increase, arising mostly from a step in solar wind density, around 15:40 UT the RBSP-ECT data show clear ULF wave modulation at the drift period spanning a very large range in energy from at least 200 keV to over 4.5 MeV. For example, at energies of around 1 MeV, clear modulation can be seen to last from at least 15:40–18:00 UT. In Fig. 5 , there is clear evidence of a modulation frequency which is energy dependent. Higher energy particles demonstrate higher frequency modulation, consistent with particle acceleration and deceleration in response to the impulse generating drift-phase bunching and hence modulations at the drift period–also known as drift echoes. Although such drift echoes have been observed before, the range in energy and the period of the response is remarkably broad and long–reaching energies ~4.5 MeV, and lasting from at least 15:40–18:00 UT. Interestingly, the 730 keV energy channel does not show any ULF flux modulation – with 180° phase change in modulation across this channel. This will be the subject of future analysis and detailed modelling. Such drift echoes can be considered equivalent to the action of an m =1 drift resonance spanning a very broad range of energies (and hence drift frequencies) in response to the broad frequency ULF response excited in the magnetosphere by the solar wind impulse. An important question is why such clear, and prevalent, ULF modulation seen for such long intervals and across such a wide range of energies by RBSP-ECT (of which this is but one example of many) was not seen with other previous satellite particle experiments? Figure 5b , which shows three channels of MagEIS histogram data with unrivalled energy resolution of around 9.6 keV, reveal the answer: phase mixing in broader energy channels would likely quickly smear out ULF modulation. In contrast to earlier observations, the ECT data (including the MagEIS histogram data in Fig. 5b ) demonstrate the richness, complexity and energy and frequency dependence of the electron radiation belt response which is being revealed by the Van Allen Probes. The period from around 15:40–16:20 UT in Fig. 5a reveals an additional very interesting coherent ULF modulation at ~5.6 mHz from around 20–450 keV. As in the LANL and CRRES data from 24 March 1991 ( Fig. 2 ), the RBSP-ECT ULF modulation also shows a clear 180° phase change with energy suggestive of a ULF wave resonant response. However, unlike the relativistic CRRES event (resonant energy ~500 keV), RBSP-ECT event suggests a resonant energy ~60 keV at apogee around L =5.5. To be resonant at the observed RBSP-ECT energy range requires a high- m wave with m ~44. RBSP-B ( L =5.9, MLT=6.7 at 16:00 UT; data not shown) was also close to apogee and east of RBSP-A; it saw modulation at similar energies, but neither as coherent nor at the same discrete frequency at RBSP-A (see Claudepierre et al. [28] for further details and analysis). Such low energy particles cannot complete entire drift transits around the Earth during the ULF wavetrain, suggesting that ULF modulation was only active very close to RBSP-A–evolution along the drift path explaining the signals seen further east at RBSP-B. Interestingly, the RBSPs were over the western CARISMA ground-based magnetometer array [29] —with RBSP-A magnetically conjugate to Dawson City. Only this station saw a clear coherent ~5.6 mHz ULF wavetrain, the same frequency as the electron flux modulation seen by the Van Allen Probes, suggesting narrow azimuthal spatial localization. Such spatial localization of ULF waves is expected for moderate- m FLRs which can be excited by energetic particles. Localized ULF waves may be excited by unstable ring current particle distributions [30] , providing a potential pathway for the ring current to drive the radiation belts [31] . Further detailed observational and modelling studies of such events are warranted [28] , motivated by the discovery and observations presented here. The results presented here show that rather than having an azimuthally symmetric structure the Van Allen belts can have significant ULF modulation fine structure which manifests itself as a function of particle energy, azimuth, L-shell and time (see Fig. 5 ). Figure 5c in particular shows a schematic of the coherent interaction between eastward drifting, relativistic Van Allen Belt electrons and ULF waves in the magnetosphere. The wave–particle interaction creates drift-phase bunched electrons which are observed as flux modulations by energetic particle detectors. Based on the observations presented here, coherent interactions with ULF waves appear to be much more important for radiation belt transport, structuring, dynamics and energization than previously thought–challenging the standard paradigm in radiation belt modelling that transport on the drift timescale is always diffusive in nature. In the future, further analyses using data from the Van Allen Probes mission will enable the relative impact of multiple plasma wave–particle acceleration and loss processes to be compared. Determining the nature of the dominant acceleration and loss processes is essential for developing more accurate physics-based space radiation forecast models. Even under the contemporaneous action of very low frequency wave acceleration, for example, as discussed by Reeves et al. [5] , additional redistribution of radiation belt flux under the action of ULF waves represents a critical element of belt dynamics. Similarly, in a broader context, our results present observational evidence for the importance of the action of coherent periodic betatron acceleration process in the dynamics of wind-driven astrophysical magnetospheres. Nowhere else in the universe is there the opportunity to observe in situ , and with such clarity, the physical nature of these collisionless processes. This can be contrasted with astrophysical studies which typically have to rely on remote sensing using electromagnetic emissions for inferences about the nature of the dominant plasmaphysical interactions. How to cite this article: Mann, I.R. et al. Discovery of the action of a geophysical synchrotron in the Earth’s Van Allen radiation belts. Nat. Commun. 4:2795 doi: 10.1038/ncomms3795 (2013).